Nanotomy-based production of transferable and dispersible graphene nanostructures of controlled shape and size Because of the edge states and quantum confinement, the shape and size of graphene nanostructures dictate their electrical, optical, magnetic and chemical properties. The current synthesis methods for graphene nanostructures do not produce large quantities of graphene nanostructures that are easily transferable to different substrates/solvents, do not produce graphene nanostructures of different and controlled shapes, or do not allow control of GN dimensions over a wide range (up to 100 nm). Here we report the production of graphene nanostructures with predetermined shapes (square, rectangle, triangle and ribbon) and controlled dimensions. This is achieved by diamond-edge-induced nanotomy (nanoscale-cutting) of graphite into graphite nanoblocks, which are then exfoliated. Our results show that the edges of the produced graphene nanostructures are straight and relatively smooth with an I D / I G of 0.22–0.28 and roughness <1 nm. Further, thin films of GN-ribbons exhibit a bandgap evolution with width reduction (0, 10 and ~35 meV for 50, 25 and 15 nm, respectively). The shape/size dependent quantum confinement in graphene nanostructures (GNs) control their electrical [1] , [2] , [3] , magnetic and optical properties [4] , [5] , [6] , [7] , [8] , [9] . Several studies have indicated that GNs with controlled structure can be incorporated into a wide variety of applications in electronics, optoelectronics and electromagnetics. However, there is a need for a process to synthesize GNs with varied, but controlled, shapes and defined size over a wide range (<100 nm), such that the GNs can be easily transferred to different substrates or dispersed in different solvents. Current top-down techniques to produce GNs include the following: lithography [5] —challenging to disperse GNs in solvents or to transfer to other substrates, low edge-smoothness, low throughput; chemical and sono-chemical methods [10] —produces uncontrolled size/shape; unzipping of carbon nanotubes (CNTs) [2] —restrictive to graphene nanoribbons (GNRs), uncontrolled size; and opening of Fullerenes [11] —produces substrate-bound circular GNs, uncontrolled shape, challenging to transfer/disperse. Bottom-up, solution-based synthetic routes for graphene quantum dots (GQDs) are based on Diels-Alder, cyclotrimerization and/or cyclodehydrogenation reactions [12] to control the GN size [13] , [14] . However, these chemistries fail for more than 100 ringed GQDs [13] , [14] , [15] , [16] , [17] . This is attributed to the challenge in the synthesis/stabilization of precursors, and to the decrease in solubility of the poly-aromatics in the synthesis solvents [12] , [18] . It is interesting to note that GNs do not share the fate of metal and semiconducting nanoparticles, which can be controllably synthesized in liquid phase via salt reduction. To enable manipulation of the electronic states in GNs, there is a need for a process to synthesize GNs of predefined shapes and dimensions. To address this challenge, here we report a process to produce nanoscale blocks of highly oriented pyrolytic graphite (HOPG) with controlled size/shape and consisting of columnar-stacked GN layers. These nanoblocks were exfoliated to produce corresponding GNs. Nanotomy process Producing nanoblocks of graphite constitutes the most plausible process for top-down processing of GNs. It is important to note that nanoscale graphite precursors of controlled shape and size have been a challenge to produce, whereas microscale blocks of graphite can be produced via lithography, as shown in the pioneering work by Ruoff et al . [19] To produce nanoscale HOPG construct, we developed a top-down strategy to cleave HOPG (ZYA grade, 0.4±0.1 mosaic spread) via diamond-edge-induced serial nanotomy. Here the diamond edge is kept perpendicular to the graphenic planes of the HOPG, which is subsequently cleaved via C–C bond stretching and crack formation in the direction of cleavage (simulation results discussed later). Depending on the desired shape/size, the HOPG is cut several times, at controlled thicknesses and in different directions, to produce GNBs of defined dimensions and shape ( Fig. 1 ; Supplementary Fig. S1 ; Supplementary Movie 1 ). Each of these GNBs consists of millions of columnar-stacked GNs with same dimensions and shape. To produce GNRs of controlled width, the GNBs were cleaved at the corresponding thickness. These GNBs were ~1 mm long×~1 mm wide. The GNB-cleavage is governed by crack-propagation (shown later), which produces relatively smooth edges. For GQDs, the GNBs were cleaved via a two-step process to control the width, length and angles, corresponding to the desired shape and size. All GNBs were subsequently exfoliated in superacid [20] and diluted in aqueous solution to produce a stable suspension of pristine GNs ( Fig. 1d,e ; Supplementary Fig. S1 ). 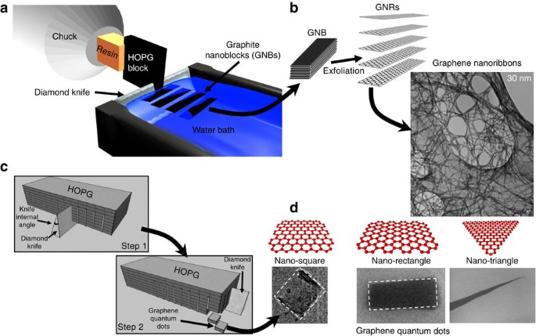Figure 1: Schematic diagram for the GN production process. (a) A descriptive sketch of the nanotomy process showing the diamond-knife-based mechanical cleaving of HOPG block to produce GNBs for GNR production. Process parameters:dr=step-size andθv=angle of cleavage. (c) Sketch of the two-step nanotomy process to produce GNBs for GQD production. (b,d) GNRs and GQDs are produced by exfoliating the corresponding GNBs in chlorosulphonic acid (superacid). TEM micrographs of 30 nm GNRs and FESEM micrographs of GQDs of different shapes (square, rectangle and triangle). Figure 1: Schematic diagram for the GN production process. ( a ) A descriptive sketch of the nanotomy process showing the diamond-knife-based mechanical cleaving of HOPG block to produce GNBs for GNR production. Process parameters: d r =step-size and θ v =angle of cleavage. ( c ) Sketch of the two-step nanotomy process to produce GNBs for GQD production. ( b , d ) GNRs and GQDs are produced by exfoliating the corresponding GNBs in chlorosulphonic acid (superacid). TEM micrographs of 30 nm GNRs and FESEM micrographs of GQDs of different shapes (square, rectangle and triangle). Full size image In a typical process, an HOPG block (SPI) is firmly mounted to the arm of the nanotome (PT-XL Microtome, Boeckeler Instruments; Supplementary Fig. S1 ) via araldite resin, which provides structural support to the HOPG block. The graphenic planes are precisely aligned perpendicular to the edge of a diamond knife (Du Pont, 45° included angle, 5° clearance angle, and 40° rake angle) with a controlled angle between the plane of the leading edge of the HOPG block and the knife axis ( θ v ) (non-zero for triangular GQDs or tapered GNRs). Then, by controlling the forward step size, d r , of the nanotome's sample arm, GNBs of controlled dimensions were cleaved serially from the parent HOPG block ( Fig. 1a,b ; Supplementary Movie 1 ). For GNRs, the GNBs were cut in a single direction and were collected in a water trough behind the diamond knife ( Supplementary Fig. S1c ). For GQDs, we coated the HOPG with wax, and then cleaved it in two directions ( Fig. 1 ). The wax provides support for the GNBs after the cuts in the first direction. Perpendicular directions resulted in square and rectangular GQDs whereas other angles resulted in triangular GQD or tapered GNR. As expected, the yield for the GNB-synthesis is 100%. A variant form of the nanotomy process has been employed by Whitesides et al . to cleave thin gold films into gold nanoparticles [21] , [22] , [23] . After the production of GNBs, they can be exfoliated via different graphene exfoliation methods [10] , [24] , [25] , [26] , [27] , [28] . To obtain unoxidized GNRs, we employ the superacid-based-exfoliation strategy (80% efficiency, Supplementary Fig. S1e ) [29] , where the superacid quenches the π – π interaction between the graphene sheets. The automated nanotome produces one HOPG cut per second. In our process, the HOPG (0.4 cm×0.4 cm×0.5 cm) is nanotomed over an area of 1×1 mm 2 and to a thickness of 5 mm. Therefore, for 20 nm square GQDs, it takes 2.7 h to produce 4×10 13 GQDs from 2.5×10 7 GNBs (each GNB has 1.6×10 6 GQDs). Thus, 1.48×10 13 GQDs can be produced per hour. Commercial nanoparticle-solutions (gold, silver, polystyrene and so on) usually come in 50 ml bottle with a concentration of 10 10 nanoparticles per ml. Thus, ~30 bottles of 50 ml GQDs solution (10 10 # per ml=112 μg ml −1 ) can be produced per hour. Similarly, for 15 nm×10 microns graphene nanoribbons, ~10 11 GNRs can be produced per hour. Hummer's acid exfoliation and pyrene carboxylic acid-based Π-intercalation exfoliation [30] were also conducted successfully. It is also important to note that the exfoliation of graphite involves sheet shearing during exfoliation, which leads to tearing; however, GNBs have smaller lateral dimensions leading to lower shear and thus less tearing. Further, the Hummer's process produces shorter GNRs due to extensive oxidative cleavage; therefore, a lower concentration of acids was used for exfoliation. To obtain GNRs with width below 10 nm, angular nanotomy of HOPG was conducted, where the diamond-knife edge was aligned parallel to the graphene surface at an angle of 3° with the perpendicular face, which led to production of 1–10 nm wide GNRs. Supplementary Fig. S4a shows a 5 nm GNR produced via this process. Structural characterization For field-emission scanning electron microscope (FESEM) and transmission electron microscope (TEM) analyses, the as-exfoliated GNs were deposited on doped silicon wafers and 400 mesh lacey carbon grids, respectively. Figures 1 and 2 show a collection of TEM images of 15, 30, 40 and 60 nm wide GNRs; 120 and 600 nm graphene ribbons; 50-nm square GQDs; 25×100 nm 2 rectangular GQDs; and 8° tapered GNRs. We also synthesized GNRs with a width of 5 nm via this process ( Supplementary Fig. S4a , top inset). It is clear that this process is versatile to control the shape and size (at 5 nm resolution) of the GNs. The standard deviation in width varies from ~1 nm to ~5 nm from batch to batch of the as-produced samples ( Supplementary Information ). Moreover, the process allows suspending the GNs (>10 8 ml −1 ) in different solvents ( Supplementary Information ). Atomic force microscopy (AFM) scans on the GNRs immobilized on silicon dioxide substrate showed several monolayer and bilayer GNRs ( Supplementary Fig. S5 ). This is consistent with the results reported by Hernandez et al . [24] for graphene suspension. The GNRs had a uniform width in the longitudinal direction, with the diffraction-pattern displaying the crystallographic signature of the honeycomb graphitic lattice ( Supplementary Information ). Further, high-resolution transmission electron microscopy (HRTEM) showed the atomic-lattice and the edge crystallography of a 15-nm GNR deposited on lacey carbon grids (SPI) ( Supplementary Fig. S6 ). We also found that Hummers method efficiently exfoliates the GNBs to produce oxidized GNs. The oxy-groups on GNs keep them stretched and stably dispersed. A dispersion of 50 nm square oxidized GQDs (GOQDs) was tested for photoluminescence. When excited at 320 nm (absorption peak), the GOQD-dispersion exhibited a PL emission at 390 nm, at which two excitation peaks were observed at 320 nm and 265 nm. A more detailed study will be published soon. 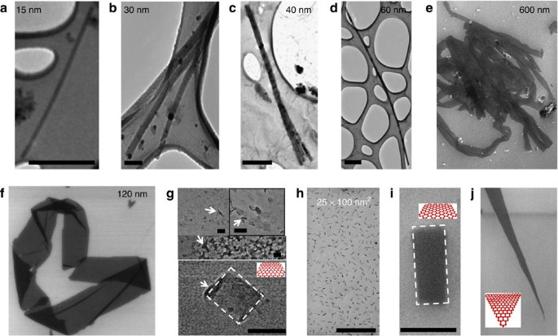Figure 2: GNRs and GQDs of controlled shape and size. TEM micrographs of GNRs of (a)w=15, (b)w=30, (c)w=40 (exfoliating), and (d)w=60 nm deposited on 400 mesh lacey carbon grids and (e) FESEM micrograph of 600 nm ribbon were obtained. (f) Electron microscope images of a 120-nm graphene ribbons (FESEM), (g) 50 nm square GQDs (FESEM), (h,i) 25×100 nm2rectangular GQDs (FESEM), and (j) 8°-angled tapered GNR (or triangular GQD) (FESEM)) were also obtained. The large densities of square and rectangular GQDs (g) showed extensive folding (white arrows). The standard deviation in width ranges from 3 to 5 nm forw~20–40 nm GNRs. This is attributed to the diameter of the knife edge=1–2 nm. (Supplementary Fig. S4for additional images). Bar sizes=(a) 250 nm, (b,g,i) 50 nm, (c,d) 500 nm, and (h) 1 μm. Figure 2: GNRs and GQDs of controlled shape and size. TEM micrographs of GNRs of ( a ) w =15, ( b ) w =30, ( c ) w =40 (exfoliating), and ( d ) w =60 nm deposited on 400 mesh lacey carbon grids and ( e ) FESEM micrograph of 600 nm ribbon were obtained. ( f ) Electron microscope images of a 120-nm graphene ribbons (FESEM), ( g ) 50 nm square GQDs (FESEM), ( h , i ) 25×100 nm 2 rectangular GQDs (FESEM), and ( j ) 8°-angled tapered GNR (or triangular GQD) (FESEM)) were also obtained. The large densities of square and rectangular GQDs ( g ) showed extensive folding (white arrows). The standard deviation in width ranges from 3 to 5 nm for w ~20–40 nm GNRs. This is attributed to the diameter of the knife edge=1–2 nm. ( Supplementary Fig. S4 for additional images). Bar sizes=( a ) 250 nm, ( b , g , i ) 50 nm, ( c , d ) 500 nm, and ( h ) 1 μm. Full size image We also probed the chemical structure of the GNRs (exfoliated via superacid) by X-ray photoelectron spectroscopy (XPS). The C-1s spectra for the GNRs showed a large sp 2 carbon peak at 284.5 eV ( Fig. 3h ). This is consistent with the earlier results reported for graphene dispersions in superacid [20] , organic and inorganic solvents [24] , [31] . The quality of the as-produced GNRs was also investigated using Raman spectroscopy (514.5 nm;<5 mW) [32] . GNRs (post-exfoliation) with widths ~15, 25 and 50 nm (confirmed by TEM images and the FESEM images) were drop-casted as films on a heavily doped n-type silicon substrate, dried in a 20 psi ultrahigh-purity (UHP) argon atmosphere and calcinated at 200 °C for 2 h in vacuum (10 −5 Torr). The I D / I G ratios were used as a measure of GNR's edge-quality [33] (relative edge roughness/defect-density, including dangling bonds and crystallographic randomness [34] ) ( Supplementary Fig. S8 ). As the laser-beam diameter was ~0.4 μm, the Raman spectrum provides the average quality of several GNRs. This also accounts for the relatively broad peaks, especially the 2D peak [35] ( Fig. 3 ). The I D / I G ratio ranges from 0.22 to 0.28 for the as-synthesized GNRs with the narrower ribbons having relatively higher I D / I G ( Fig. 3a,c,e ). On comparing with the literature data on GNRs with similar dimensions, these values are close to that reported for GNRs produced via sonochemical unzipping of CNTs [10] and are significantly lower than that for lithography and other GNR production techniques ( Fig. 3g ) [1] , [2] , [3] , [34] . This indicates relatively smooth edges of the produced GNRs. Further, conformal Raman mapping of the individual bilayer GNRs, immobilized on SiO 2 substrate, was also recorded. The average I D / I G ratio for the w ~15 nm GNRs was between 0.25 and 0.4 (see Supplementary Fig. S8 ), comparable to the GNRs of similar widths synthesized by sonochemical unzipping of CNTs [10] and much lower than those produced by lithographic methods ( I D / I G ~1.5) or oxidative unzipping of CNTs ( I D / I G ~1). Because the I D / I G ratio increases with the lattice defect, the overall low ratio indicates good quality GNs [33] . 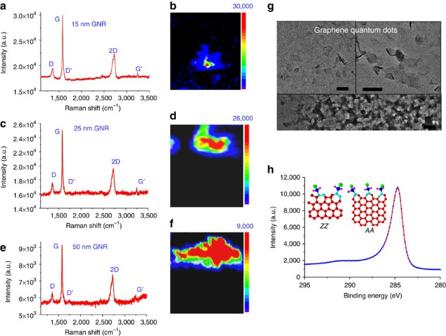Figure 3: Raman and XPS spectra of the GNRs. (a,c,e) Raman spectra and (b,d,f) G-band scans of thew=15 nm (a,b),w=25 nm (c,d) andw=50 nm (e,f) GNRs show lowID/IGratios. As expected, narrower ribbons exhibited higherID/IGbecause of higher percentage of edges. TheID/IGratios were 0.28 (a), 0.24 (b) and 0.22 (c) for 15 nm, 25 nm and 50 nm GNRs; and theI2D/IGratios were 1.25 (a), 1.04 (b) and 1.21 (c), respectively. (g) FESEM image of large quantities of 50 nm, squared GQDs. (h) Typical XPS spectra for the C 1 s-binding energies of the GNRs showing the sp2carbon peak at 284.5 eV with high-percentage carbon >98%. High-resolution XPS scans for S 2p-binding energies (seeSupplementary InformationandSupplementary Fig. S7) showed traces of sulphur (~0.92%). Inset shows the chemical structure of a probable edge-sulphonation-chemistry on the armchair (AA) and zigzag (ZZ) GNR edges24. Figure 3: Raman and XPS spectra of the GNRs. ( a , c , e ) Raman spectra and ( b , d , f ) G-band scans of the w =15 nm ( a , b ), w =25 nm ( c , d ) and w =50 nm ( e , f ) GNRs show low I D / I G ratios. As expected, narrower ribbons exhibited higher I D / I G because of higher percentage of edges. The I D / I G ratios were 0.28 ( a ), 0.24 (b) and 0.22 (c) for 15 nm, 25 nm and 50 nm GNRs; and the I 2D / I G ratios were 1.25 (a), 1.04 (b) and 1.21 (c), respectively. ( g ) FESEM image of large quantities of 50 nm, squared GQDs. ( h ) Typical XPS spectra for the C 1 s-binding energies of the GNRs showing the sp 2 carbon peak at 284.5 eV with high-percentage carbon >98%. High-resolution XPS scans for S 2p-binding energies (see Supplementary Information and Supplementary Fig. S7 ) showed traces of sulphur (~0.92%). Inset shows the chemical structure of a probable edge-sulphonation-chemistry on the armchair (AA) and zigzag (ZZ) GNR edges [24] . Full size image Molecular dynamics simulations The nanotomy process creates high local tensile (in direction perpendicular to cutting) and compressive (in the direction of cutting) stresses at the point of contact between the HOPG and the diamond knife. To understand the mechanism of lattice cleavage and the evolution of the edge structure of the GNs produced, we performed molecular dynamics (MD) simulations for the diamond-nanotomy process ( Fig. 4a,b ; Supplementary Methods ), where monolayer and multilayer graphene sheets of finite size are constrained at the sides perpendicular to the cutting direction and cleaved afterwards by a diamond nanorod ( Fig. 4a,b ). Our simulation results show that high tensile stress ( Fig. 4a ; Supplementary Fig. S14a–c ) at the knife edge leads to stretching and breaking of the carbon–carbon sp 2 bonds ( Supplementary Fig. S13a shows the cleaving of a GNB from HOPG). As a result, the crack propagates along the cutting direction and globally cleaves straight edges, no matter how the lattice orientation of graphene aligns with the cutting direction ( Fig. 4b ; Supplementary Fig. S14 ). However, at the crack front, the atomic structures of cleaved graphene edges are locally defined by the pattern of breaking bonds under the loading condition and their reconstruction under specific chemical environment ( Fig. 4c ). As the cleavage occurs because of tearing under tensile stress, additional MD simulations were also carried out for graphene sheets tearing under tensile stress [36] , [37] , [38] . This is similar to the local tensile stress experienced by HOPG in the direction perpendicular to the cutting-direction. We observe that the carbon–carbon sp 2 bonds cleave and form cracks oriented perpendicular to the tension load, and these cracks primarily consist of zigzag edges at atomistic scale ( Figs 4e and 13b,c) [38] . As recently predicted, these zigzag edges readily rearrange into energetically more favourable structures such as Stone-Wales defects [39] ( Fig. 4c ), owing to the instability of dangling bonds on graphene edges. Density functional theory-based calculations show that reconstructed zigzag edges feature the lowest energy within several explored edges, followed by pristine, reconstructed armchair, and pristine zigzag edges [40] . Graphene edges reconstruct during and after the fracturing process, which can be very complicated in oxidative or hydrogen-rich environments. Also shown in the simulation results, the cleaving process yields dangling carbon bonds with an average roughness less than 1 nm. This combined effect on the fracturing pattern, from both the stress field induced and edge reconstruction, defines straight and clean edges that are interesting for electronic applications. To verify the MD results, we also conducted the HRTEM imaging of the GN edges. 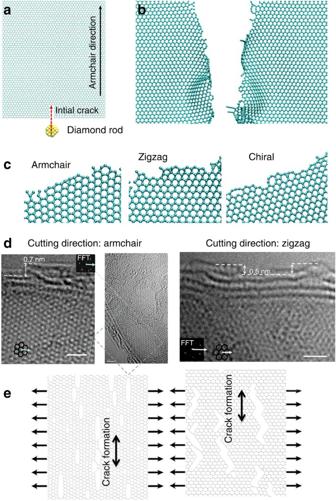Figure 4: MD simulations representing the mechanism of cutting and the edge structure. (a) The initial set-up of the simulation consists of a graphene sheet and a diamond rod. (b) After the cutting process (along the armchair orientation of a graphene sheet), the simulation shows that the edge is straight and along the direction of cutting. (c) The zoomed-in images of the carbon-atoms at the edge (for cutting along armchair, zigzag and chiral or mixing armchair-zigzag orientations) show that the edge roughness is less than 1 nm: a consequence of the dangling bonds created during nanotomy. This is compared with an HRTEM image of a 4-layered GQD, which shows a relatively smooth edge. (d) HRTEM micrographs showing the edge crystallography of two GNRs, one nanotomed in the zigzag and the other in the armchair direction. The edge roughness for zigzag is lower than that of the armchair direction. Bar=1 nm. (e) Tensile simulations were conducted to study the graphene sheet under tensile stress along its armchair and zigzag chain directions, respectively. In both cases, zigzag-edged cracks are nucleated perpendicular to the loading direction. The typical HRTEM images are shown in Figure 4d . The edges shown are for GNs nanotomed in the zigzag and armchair directions, respectively. As predicted by MD, the edges for the zigzag nanotomy direction are smoother than those for the armchair direction. The edges roughness (~0.5–0.7 nm) is similar to that for GNR produced via unzipping carbon nanotubes [41] , as also suggested by Raman data. Figure 4: MD simulations representing the mechanism of cutting and the edge structure. ( a ) The initial set-up of the simulation consists of a graphene sheet and a diamond rod. ( b ) After the cutting process (along the armchair orientation of a graphene sheet), the simulation shows that the edge is straight and along the direction of cutting. ( c ) The zoomed-in images of the carbon-atoms at the edge (for cutting along armchair, zigzag and chiral or mixing armchair-zigzag orientations) show that the edge roughness is less than 1 nm: a consequence of the dangling bonds created during nanotomy. This is compared with an HRTEM image of a 4-layered GQD, which shows a relatively smooth edge. ( d ) HRTEM micrographs showing the edge crystallography of two GNRs, one nanotomed in the zigzag and the other in the armchair direction. The edge roughness for zigzag is lower than that of the armchair direction. Bar=1 nm. ( e ) Tensile simulations were conducted to study the graphene sheet under tensile stress along its armchair and zigzag chain directions, respectively. In both cases, zigzag-edged cracks are nucleated perpendicular to the loading direction. Full size image At high cutting speeds, more defects will be created, as relaxation of edge structures is limited. Therefore, faster cleaving speed (that is, a higher specimen-arm velocity) must increase the roughness of the edges. This was verified by mapping the average Raman I D / I G ratio with the cleaving speed. I D / I G ratio=~0.83 for fast (1 mm s −1 ) compared with ~0.22 for slow (0.4 mm s −1 ) for w ~15 nm GNRs. Therefore, reducing the cutting speeds further will make the edges smoother. Unlike sublimation and chemical etching [42] , [43] , [44] , where the edge-dependent reactive energy barrier controls the edge shape, the nanotomy process yields a controlled edge-direction, which can be completely controlled to produce different shapes of GNs. Electrical characterization As the width of a GNR governs its bandgap ( 1/ w ), thin films of GNRs must exhibit width-dependent bandgap. We leveraged the width-controllability and the high-productivity of this process to study this effect for thin GNR-films. We investigated 50-nm thick films of GNRs with widths ( w ) of ~50, 25 and 15 nm ( Fig. 5f ) fabricated via filtering their dilute dispersions (~0.2 mg l −1 ) on polycarbonate filters ( Fig. 5b,c inset; Supplementary Fig. S10 ). FESEM surveys and AFM scans (typical film surfaces shown in Fig. 5e,f ) on these films showed a uniformly smooth and homogenous surface topography without local aggregates. Sheet resistance of the GNR-films, as determined from the four-point probe measurements, was between 2.2 and 5.1 MΩ/□ with no apparent dependence on the width of the constituting GNRs (3 devices were tested for each width). 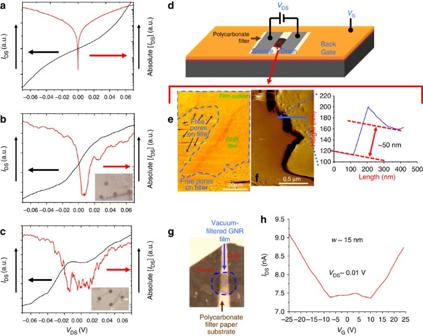Figure 5: Electrical characterization of thin GNR-films. (a,b,c) Typical high vacuum (10−5Torr), low temperature (80 K)IDSversusVDSmeasurements (linear scale) of thew~50, ~25 and ~15 nm GNR-film devices and the corresponding absolute (IDS) versusVDScurves (logarithmic scale) show nonlinear transport behaviour (panelsdandg: schematic diagram of the device and a typical optical image of the device). The edges of the bandgap were determined from the sharp current increase in the log-scale curve (red). Owing to the relatively large channel lengths of the GNR film-devices, the channel-length dependence of the nonlinear transport gap is expected to be negligible. A bandgap scaling with GNR width was observed: the bandgaps for the as-produced films withw=~50, 25 and 15 nm GNRs were ~0 meV, ~10 meV and ~35 meV, respectively (this is appropriate because panelhshows that the conductivity is well centred around zero volt bias). Insets of panelsbandcshow an optical image of the respective GNR films on the polycarbonate filter after drying. After deposition of electrodes, these polycarbonate sheets were deposited on gold substrates as shown in paneld. (e) FESEM image of a typical GNR film (as shownw~15 nm GNR film) on a polycarbonate filter substrate. (f) Tapping-mode AFM (left inset) image of the GNR film shows a typical thickness of ~50 nm (right inset). (h) A 15-nm GNR film at 10 mV (VDS), gated with voltage in the ±25 V range exhibits a semiconducting behaviour with symmetric hole and electron densities. The electron mobility measured from transconductance is ~20 cm2V−1s−1. Figure 5: Electrical characterization of thin GNR-films. ( a , b , c ) Typical high vacuum (10 −5 Torr), low temperature (80 K) I DS versus V DS measurements (linear scale) of the w ~50, ~25 and ~15 nm GNR-film devices and the corresponding absolute ( I DS ) versus V DS curves (logarithmic scale) show nonlinear transport behaviour (panels d and g : schematic diagram of the device and a typical optical image of the device). The edges of the bandgap were determined from the sharp current increase in the log-scale curve (red). Owing to the relatively large channel lengths of the GNR film-devices, the channel-length dependence of the nonlinear transport gap is expected to be negligible. A bandgap scaling with GNR width was observed: the bandgaps for the as-produced films with w= ~50, 25 and 15 nm GNRs were ~0 meV, ~10 meV and ~35 meV, respectively (this is appropriate because panel h shows that the conductivity is well centred around zero volt bias). Insets of panels b and c show an optical image of the respective GNR films on the polycarbonate filter after drying. After deposition of electrodes, these polycarbonate sheets were deposited on gold substrates as shown in panel d . ( e ) FESEM image of a typical GNR film (as shown w ~15 nm GNR film) on a polycarbonate filter substrate. ( f ) Tapping-mode AFM (left inset) image of the GNR film shows a typical thickness of ~50 nm (right inset). ( h ) A 15-nm GNR film at 10 mV ( V DS ), gated with voltage in the ±25 V range exhibits a semiconducting behaviour with symmetric hole and electron densities. The electron mobility measured from transconductance is ~20 cm 2 V −1 s −1 . Full size image The GNR-film-based field effect transistors were fabricated by sputter-coating gold–palladium (3:2) source and drain electrodes on the GNR films on the polycarbonate substrate, using resist-free shadow masking (~200 μm channel length and ~400 μm channel width) (Methods and Supplementary Methods ) ( Fig. 5g ). In addition to the absence of any short-channel effects, the relatively long-channel dimensions ensured bulk-limited transport with insignificant influence on the contact-characteristics [45] , [46] . High-vacuum (10 −5 Torr), low-temperature (80 K=6.7 meV) current-voltage characteristics ( I DS versus V DS ) of the w ~50, 25 and 15 nm GNR films at zero gate ( V G =0) and near-zero source-drain bias ( V DS ) exhibited an increase in semiconductor character with reducing width. The bandgap, determined by the edges of the steep logarithmic increase of current, scaled inversely with the GNR width: ~0 meV for w ~50 nm, ~10 meV for w ~25 nm and ~35 meV for w ~15 nm ( Fig. 5a–c ) [45] , [47] . Further, Figure 5h shows that the minimum conductivity is centred at zero gate voltage ( w ~25 nm GNR film); thus, validating the bandgap measurement at 0 V gate potential. Because of the relatively long channel lengths in the GNR film devices, the channel-length dependence of the nonlinear bandgap [47] is expected to be inconsequential. We attribute the barriers to quantum confinement in the constituent GNRs. Further, the low bandgap attests to the relatively low level of edge distortion in these GNRs. We confirmed the above-mentioned results by analysing the temperature-dependent transport behaviour for w =15 and w =25 nm GNR-films [48] . The transport properties were analysed via Arrhenius fitting of the OFF currents (zero gate bias) at higher temperatures (25 meV> T >12.5 meV (150 K)): The average thermal activation energies, E a were ~6 meV and ~30 meV for w ~25 and 15 nm GNR films, comparable to their bandgap determined from nonlinear transport characteristics. At lower temperatures ( T < T * (transition temperature=12.5 meV for 15 nm GNRs)), the OFF currents deviated from the simple activation behaviour, decreasing more slowly, a characteristic of variable range hopping behaviour, expected because of the large density of overlapping GNRs in the film [49] . We fit the variable range hopping model given by, for the conductivity at low temperature. For both γ =1/3 and γ =1/4, similar standard deviations were obtained suggesting hopping in 2 and 3 dimensions, indicating transport through randomly distributed scattering sites at the overlays of the GNRs and through multiple layers [49] . As the transport in a film with a randomly overlaying GNRs is similar to that through a heavily distorted GNR, we calculated the average width of a distorted GNR, which would have a transition temperature ( T *) of 12.5 meV (the T * we measured for 15 nm GNR). This was achieved via the correlation developed by Han et al . ( , where =347 meV) [47] . Consistently, the width from this correlation is 15.9 nm, similar to the width of the GNRs used in the film (15 nm). For electrical gating, the gold surface was used as bottom gate and polycarbonate as the dielectric ( ~2.9) (Methods and Supplementary Methods ) ( Fig. 4d ). In-air charge-transfer characteristics of the devices showed n-type doping attributed to physisorbed chemical species ( Supplementary Fig. S11 ). This was consistent with the close to unity values of I 2D / I G and red shift of 2D peak in the Raman spectra [50] ( Fig. 3a,c,e ). The devices were electrically annealed in vacuum (10 −5 Torr) to remove adsorbates (as described in ref. 51 ), resulting in the recovery of the ambipolar transfer characteristics with symmetric electron and hole transports ( Supplementary Fig. S11 ). The carrier mobilities ranged from 20–130 cm 2 V −1 s −1 for the GNR-films ( Supplementary Information ). The overall low mobilities, as compared with single GNR [34] , are attributed to carrier scattering at GNRs' overlapping junctions and three-dimensional transport over large channel length. GNs were synthesized, via a versatile nanotomy process, with high structural control (shapes: squares, rectangles, ribbons and triangles; and size: adjusted at 5 nm resolution) and colloidal monodispersivity. The GNs are exfoliated from GNBs produced via nanotomy of HOPG. This highly versatile process can produce a variety of GN structures. Further, the Raman and the HRTEM measurement show that the GNs had relatively smooth edges; while the MD simulations and HRTEM micrographs show that the edges are predominantly zigzag. Our electrical studies show evolution of bandgap of thin GN films with GNR's width. We envision that this versatile process can provide access to a wide variety of GNs at large densities (on substrates or as dispersions) for development of fundamental optical/electrical/structural correlations and novel applications. Further, the nanotomy process may be applied to other 2D nanomaterials (BN, MoS 2 and NbSe 2 ) to produce unique 2D nanostructures, which can significantly expand the scope of their applications and fundamental studies. Preparation of GNRs Cleavage of HOPG: A 7×7×1 mm 3 HOPG block (ZYA Grade, SPI) was affixed onto a cuboidal piece of hardened araldite resin, with an orientation as shown in Figure 1 (also see Supplementary Fig. S1 ). The resin-HOPG ensemble was allowed to dry at room temperature for several days before being mounted onto the nanotome sample chuck, as shown in Supplementary Figs S1 and S2 . The chuck was then mounted onto the nanotome and bolted to position on the sample arm. The diamond knife was then mounted on the nanotome with a 5° clearance angle and 40° rake angle (see Supplementary Methods for a detailed mounting procedure). Subsequently, assiduous alignment of the cutting face of the HOPG was carried out with respect to the knife (at θ v =0°) by following the three-step procedure described by Xu et al . [52] (see Supplementary Methods for details). The knife boat was filled with de-ionized (DI) water and the level adjusted by the water pump ( Supplementary Fig. S2 ) so as to have an angle of contact of 30–50° with the back of the knife edge as shown in Figure 1a . With a pre-determined sample-forward step-size ( d r ) and a specimen-arm speed of 0.4 mm s −1 , the HOPG block was cleaved repeatedly to obtain the GNBs ( Supplementary Fig. S1c and Supplementary Movie 1 ). The cleaved GNBs were collected from the knife boat. The GNBs in water was collected in clean tubes ( Supplementary Fig. S1d ) and heated at 100 °C under an UHP argon atmosphere (20 psi) for 1 h to evaporate all the water to obtain dry GNBs. Because of the importance of the sample alignment for high-quality cleaving, and to achieve best results, we used a higher d r in the beginning of the cleavage process to shape the HOPG block before proceeding onto finer cleavage steps (the initial samples were discarded). The process for GQDs is explained in more detail in Supplementary Document . Mounting/aligning the diamond knife The stage LEDs of the nanotome were switched on, while the dome light was kept off to enhance the shadows, which were used in the alignment procedure. The sample arm containing the HOPG block was parked at the same height as that of the diamond knife edge using a handwheel. While viewing through the stereoscope, the knife-stage was moved forward closer to the HOPG block edge, first within a few mm using the course adjustment knob and then closer (a few hundred microns) using the fine adjustment knob. Then, the following three-step process was employed to align the knife edge with respect to the HOPG cutting face. Alignment of the bottom edge of HOPG block parallel to the edge of the knife: The HOPG block was slowly moved past the knife edge back-and-forth (using the handwheel), while the shadow was observed that appears at the bottom of the cutting face of HOPG and disappears at the top. If the top and the bottom edges of the HOPG are parallel to the knife edge, then the shadow should first appear at the bottom of the face, move across the entire length and disappear at the top of the face. If the shadow appears at the lower edge of one side of the HOPG block before the other, then the cutting face is not parallel. The alignment of the HOPG block was adjusted using the specimen rotation alignment knob until the shadow appears evenly. Alignment of knife edge parallel to the block face across the width of block: The HOPG block was moved past the knife back-and-forth slowly using the handwheel, while observing the height of the reflection across the width of the cutting face. The reflection should be of uniform height across the whole length of the cutting face of the block. If it was higher on one side than the other, the knife alignment was changed using the stage rotation adjustment knobs until height uniformity was achieved. Alignment of the HOPG cutting face with knife edge along its whole length: The HOPG block was moved past the knife edge back-and-forth slowly using the handwheel, while observing the shadow formed at the cutting face of the HOPG. The shadow is expected to maintain the same height all along the length of the face of HOPG. If it is not, then the specimen arc rotation alignment knob was used to achieve height uniformity. During all the above alignment steps, extreme caution should be taken so as not to bump into the diamond knife edge. The diamond knife edge is very fragile to lateral stresses and extreme care should be taken while handling it at all times. Exfoliation of the GNBs The dried GNBs in glass vials were dispersed in 5 ml of >99% chlorosulphonic acid inside a glove box (<1 p.p.m. water vapour, <1 p.p.m. oxygen). The vials were subsequently placed in a shaker (inside the glove box) for ~8 h at room temperature and the exfoliation process was allowed to run to completion, inferred by dark black colour of the suspension phase with no solid residue. For characterization purposes, the GNR suspension was quenched in DI water (1:200) as per the procedure described by Behabtu et al . [20] . Fabrication of flexible pristine GNR films via vacuum-filtration 0.1 ml of the superacid-dispersed pristine GNRs was quenched in 20 ml of DI water to produce a colloidal suspension of exfoliated pristine GNRs in DI water (conc. ~0.2 mg l −1 ). Thin, flexible pristine GNR films were fabricated via vacuum filtration of water-quenched samples of pristine GNRs onto polycarbonate filters (2-inch diameter, 600-nm pore size, SPI), followed by drying in an argon atmosphere at room temperature for 2 days. Because of the use of a Büchner funnel in the filtration process, we obtained several GNR films, each having a dimension similar to the pores on the funnel (~0.4 mm in diameter). Owing to the high aspect ratio of the GNRs ( w ~15–50 nm compared with the 600-nm pore size of the filter), several layers of GNRs need to come together to block a single pore. This is different from the graphene/GO film filtration where a single sheet blocks the pore. This blockage of a pore is expected to start the deposition process by enhancing the permeation through the adjacent pore until it is clogged by the GNRs, and hence continuing until most of the pores are clogged. The average thickness of the GNR films was found to be ~50 nm. This is in contrast to the much larger GO films, where 3–5 layers (corresponding to 4–5 nm) are typical. Characterization The samples for the FESEM, XPS and Raman spectroscopy were fabricated by immobilizing the quenched GNRs via drop-casting on freshly cleaned n-type silicon wafers (University Wafers) and drying in an 20 psi UHP Ar atmosphere followed by annealing at 200 °C in vacuum (base pressure of 10 −5 Torr) for 2 h. Silicon wafers were cleaned with organic solvents (acetone and isopropanol) followed by native oxide etching with a solution of H 2 O:HF (10:1), followed by washing with isopropanol. FESEM imaging was carried out in a NovaNano FESEM, or Leo 1550 FESEM at University of Kansas (KU). XPS was carried out in a Perkin Elmer XPS. Raman spectroscopic analyses were carried out in a Renishaw InVia microRaman spectroscope equipped with a 514.5-nm laser line using a ×100 objective (NA 0.9). The samples for TEM imaging were fabricated by dipping the lacey carbon 400 mesh grids (SPI) in the freshly quenched GNR solution and drying. TEM imaging was carried out on a Philips CM 100 TEM or on a 200 kV Field-Emission TEM (at KU). The HRTEM images were obtained on a 300 kV aberration-corrected TEM (FEI Titan). Characterization of GNR film by AFM and FESEM For AFM and FESEM analysis of the GNR film, the polycarbonate filter containing the GNR-film was transferred on a freshly cleaned silicon wafer and clamped down using conductive carbon paint. FESEM imaging was carried out using the beam deceleration feature of the FEI NovaNANO FESEM with landing voltages of <1 KV. AFM imaging was carried out in tapping-mode using the EasyScan 2 AFM system from NanoScience Instruments Inc. Fabrication of thin-film pristine GNR devices GNR films on polycarbonate filter substrate were directly used for device fabrication. 0.2-mm wide polyethylene strips were used as shadow mask (to define the channel), whereas source and drain Au:Pd (3:2) electrodes were deposited via sputtering. Then, the mask was removed and the sample checked under an optical microscope to ensure proper deposition of electrodes and channel integrity. For back-gated electrical studies, the film (with source and drain deposited) was immobilized mechanically, using a polydimethylsiloxane stamp on a gold-coated silicon dioxide wafer. Here the polycarbonate substrate acts as the gate oxide, and the gold coating on the wafer acts as the back gate. Electrical characterization was carried out in a Janis ST100 cryostat connected to a turbomolecular pump and a liquid nitrogen line. How to cite this article: Mohanty, N. et al . Nanotomy-based production of transferable and dispersible graphene nanostructures of controlled shape and size. Nat. Commun. 3:844 doi: 10.1038/ncomms1834 (2012).